Observation of the intrinsic bandgap behaviour in as-grown epitaxial twisted graphene Twisted graphene is of particular interest due to several intriguing characteristics, such as its the Fermi velocity, van Hove singularities and electronic localization. Theoretical studies recently suggested the possible bandgap opening and tuning. Here, we report a novel approach to producing epitaxial twisted graphene on SiC (0001) and the observation of its intrinsic bandgap behaviour. The direct deposition of C 60 on pre-grown graphene layers results in few-layer twisted graphene confirmed by angular resolved photoemission spectroscopy and Raman analysis. The strong enhanced G band in Raman and sp 3 bonding characteristic in X-ray photoemission spectroscopy suggests the existence of interlayer interaction between adjacent graphene layers. The interlayer spacing between graphene layers measured by transmission electron microscopy is 0.352±0.012 nm. Thermal activation behaviour and nonlinear current–voltage characteristics conclude that an intrinsic bandgap is opened in twisted graphene. Low sheet resistance (~160 Ω□ −1 at 10 K) and high mobility (~2,000 cm 2 V −1 s −1 at 10 K) are observed. The rotational stacking of graphene layers alters their electronic characteristics resulting in novel and rich physics [1] , [2] , [3] , [4] , [5] , [6] , [7] , [8] . Bernal (AB)-stacked graphene rotated by 60° between adjacent layers is well understood and its electronic properties are radically different from single-layer graphene (SLG). Bernal-stacked graphene shows quadratic energy–momentum dispersion due to strong interlayer interaction and a bandgap opening due to symmetry breaking. Twisted graphene (TG) rotated by an arbitrary angle is commonly found in graphene grown on metals [3] , [9] , [10] , C-face SiC [11] or bulk graphite surfaces [12] , [13] , and is still under intensive study to identify its properties. Ab initio calculations showed that the Dirac cones and Fermi velocity of each layer preserved those of SLG due to decoupling between layers [14] . A full-tight binding calculation showed a reduction of the Fermi velocity due to interlayer interaction [2] . For TG with small twist angles ( θ <15°), the experimental studies showed [1] , [3] , [6] , [9] that the Dirac cones for each layer persist but van Hove singularities are present due to the interlayer interaction. For large twist angles, the twisted layers effectively de-couple from each other and become indistinguishable from SLG [7] . However, several theoretical reports have recently predicted the existence of coupling between large-angle twisted layers. Mele [8] predicted that the Dirac cones of TG are directly coupled across any commensurate rotational fault. The even state under sublattice exchange provides the bandgap in TG, while the odd symmetry has two massive graphene band structures. The bandgap opening in TG was also predicted by Muniz and Maroudas [4] , [5] . They proposed that fullerene superlattices are formed due to interlayer covalent C–C sp 3 bonding and cause the bandgap opening in TG. The bandgap opening in graphene has been intensively studied to utilize its extraordinary properties in practical two-dimensional (2D) nano device application and was only achieved by ex situ modification of graphene band structures, such as external gating structure, molecular doping and fabrication of graphene nano ribbon structures which have several drawbacks such as the requirement of ex situ processing steps and complex 2D device structures. Therefore, the bandgap opening method eliminating ex situ processing is highly desirable, which allows the direct adaption of state of the art Si technology. Here, we present evidence that direct growth by carbon source molecular beam epitaxy (CMBE) with C 60 molecular on pre-grown template graphene results in the twisting in graphene layers and the as-grown epitaxial twist graphene exhibits the tunable bandgap opening through the concentration variation of sp 3 interlayer C–C bonds. We previously reported the formation of an intrinsic gap in this stacked graphene [15] , but here we show that the bandgap is most likely due to fullerene superlattice and interlayer sp 3 C–C bonding in TG suggested by Muniz and Maroudas [4] , [5] . Sample growth and characterization The epitaxial TG layers were grown by the direct deposition of C 60 on top of pre-grown graphene (henceforth called the template) by CMBE on Si-face SiC. The graphene templates were grown by both CMBE using a heated graphite filament (GF) carbon source and by thermal decomposition (TD) of the SiC substrate. Angular resolved photoemission spectroscopy (ARPES) measurements on these stacked C 60 grown graphene/template graphene samples confirms that the hexagonal unit cells have an azimuthal offset angle of ~30° to each other. Transmission electron microscopy (TEM) measurements show that the interlayer spacing of the grown graphene layers is 0.352±0.012 nm, which is larger than that of coupled (Bernal-stacked) graphene layers (0.335 nm). Raman measurements indicate a significantly enhanced G band, a 2D peak shift and a narrowing of the 2D FWHM, which is typical in interacting TG layers [16] . X-ray photoemission spectroscopy (XPS) measurements show the existence of sp 3 carbon bonding as well as sp 2 bonded graphene structure. I – V measurements show nonlinear characteristics and Hall measurements demonstrate activation behaviour of the carrier concentration and conductance, which is typical of gapped semiconductors. They show low sheet resistance (~160 Ω□ −1 at 10 K) and high mobility (~2,000 cm 2 V −1 s −1 at 10 K). Atomic simulations of graphene growth using density functional tight binding method demonstrate stable sp 3 C–C bonds interconnecting graphene layers, and show that vacancy defects in template graphene lead to sp 3 hybridized carbon formation. Various defect states are speculated to be involved in the formation of sp 3 hybridized carbons during growth. Atomic simulations using density functional tight binding method are used to demonstrate possible growth situations where vacancy defects leads to sp 3 hybridized carbon formations interconnecting layers of graphene-like films. Stacking order in C 60 /GF FLG We have performed ARPES measurements to analyse the stacking of C 60 /GF FLG. 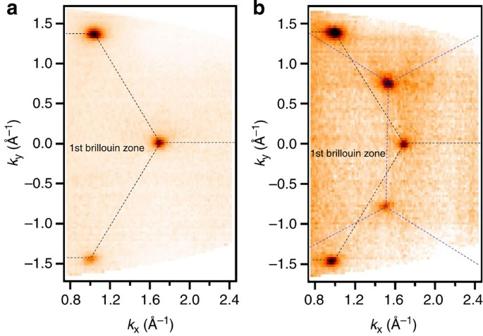Figure 1: ARPES analysis of twisted graphene. The constant energy map at the Fermi energy from ARPES measurements for (a) template graphene and (b) graphene grown by C60deposition, measured with photons of 50 eV. The template graphene shows point-like Fermi surfaces at each corner of the first Brillouin zone (BZ) of graphene denoted by black-dashed lines. The graphene grown by C60deposition shows an additional honeycomb shape denoted by blue-dashed lines, which is rotated by ~30 degrees with respect to that of template graphene. Figure 1 shows the Fermi surface map for a GF template sample ( Fig. 1a ) and a C 60 /GF few-layer graphene (FLG) structure ( Fig. 1b ). The GF template ( Fig. 1a ) shows the point-like Fermi surface at each corner of the graphene Brillouin zone. For the C 60 /GF FLG sample, however, two hexagonal unit cells rotated by ~30° to each other were observed ( Fig. 1b ). This suggests that C 60 deposition results in graphene layers that do not follow the stacking order of the underlying template but rather gives 30° rotated stacking on top of it. We note that C 60 CMBE directly on SiC often results in Bernal-stacked FLG [17] . Figure 1: ARPES analysis of twisted graphene. The constant energy map at the Fermi energy from ARPES measurements for ( a ) template graphene and ( b ) graphene grown by C 60 deposition, measured with photons of 50 eV. The template graphene shows point-like Fermi surfaces at each corner of the first Brillouin zone (BZ) of graphene denoted by black-dashed lines. The graphene grown by C 60 deposition shows an additional honeycomb shape denoted by blue-dashed lines, which is rotated by ~30 degrees with respect to that of template graphene. Full size image High-resolution cross-sectional TEM analysis The graphene interlayer distance depends on its stacking orientation. AA- and AB-stacked graphene have 3.495 and 3.35 Å (ref. 18 ), respectively. In addition, graphene on C-face SiC, which has a ~30° twist angle between adjacent layers, has a 3.368 Å interlayer distance [19] . TEM characterization of the graphene layers was performed using an aberration corrected (image) Titan 80–300 TEM operated at an accelerating voltage of 80 kV. Cross-sectional samples for TEM observations were prepared by conventional ion-milling, with the samples mounted on a liquid nitrogen-cooled cryo-stage. For this study, the sample was grown by GF CMBE for 10 min at 1,300 °C, followed by the C 60 deposition for 30 min. at 1,400 °C. 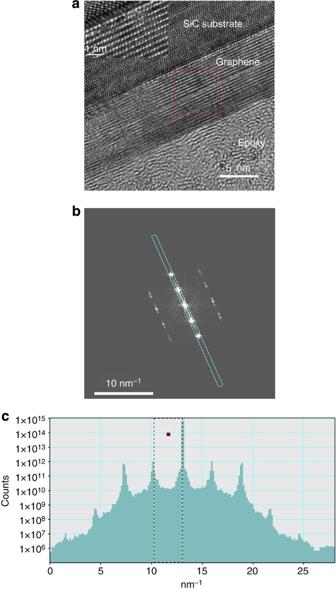Figure 2: TEM cross-section image and Fourier image analysis. (a) TEM image of graphene layers on a 6H-SiC substrate. The red square indicates the region chosen for digital Fourier image analysis. (b) Power spectrum of region within the red square ina. (c) Line profile along the marked region inb. The dashed lines identifying the maxima incare 2.81 nm−1apart, corresponding to a spacing of 0.356 nm. Figure 2a is a high-resolution TEM image of the overall structure, showing the individual graphene layers and an abrupt SiC/graphene interface. The region within the graphene layers corresponding to the change in C source is also clearly revealed. The average interlayer spacing was determined by digital Fourier image analysis, based on a measurement of the distance between the relevant maxima in the power spectrum of a region within the graphene layers. Figure 2b is the power spectrum of the region within the graphene layers indicated in Fig. 2a , where the maxima corresponding to interlayer spacing along the [0001] are observed. Figure 2c is an intensity profile along the maxima from which the average interlayer spacing was determined. It is worth noting that these measurements were calibrated with reference to the [0002] spacing of the SiC substrate, which was determined using the same procedure from a region far away from the interface. On the basis of these measurements, the average interlayer spacing was determined to be 3.52±0.012 Å. The observed interlayer distance is larger than that of strongly coupled Bernal-stacked graphene layers (~3.35 Å) [18] , [20] , and graphene on C-face SiC (3.368 Å) [19] . Although the twist angle of C 60 /GF is the same as that of graphene on C-face SiC, the interlayer spacing is larger than that of the graphene on C-face SiC. Figure 2: TEM cross-section image and Fourier image analysis. ( a ) TEM image of graphene layers on a 6H-SiC substrate. The red square indicates the region chosen for digital Fourier image analysis. ( b ) Power spectrum of region within the red square in a . ( c ) Line profile along the marked region in b . The dashed lines identifying the maxima in c are 2.81 nm −1 apart, corresponding to a spacing of 0.356 nm. 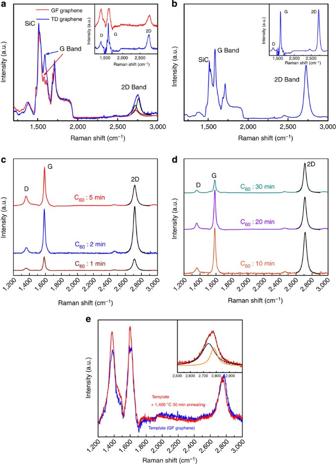Figure 3: Raman studies for graphene layer stacking order. Raman spectra of TD template (blue colour ina) and C60/TD FLG sample (red colour ina). inset) spectrum with SiC signal subtracted. 2D band of TD template has two Lorentzian components (black coloured curves), indicating Bernal stacking structure. (b) C60/TD FLG spectrum is composed of a single Lorentzian peak, indicating non-Bernal-stacked structure. Inset) spectrum with SiC signal subtracted. (c,d) Variation of Raman C60/GF FLG spectra as a function of C60deposition time. A single Lorentzian 2D band was observed for all samples studied. Black solid curves represent the fitted curve. (e) Comparison of GF template before and after thermal annealing for 30 min at 1,400 °C. Inset) curve fitting of 2D band of GF template sample. Full size image Raman studies of twisted graphene Figure 3 shows the Raman spectra for two different template types (TD and GF graphene) and FLG after C 60 deposition on them. As seen in Fig. 3a , the G band intensity of the TD (blue spectrum) and GF (red spectrum) template is smaller than that of the SiC Raman signal and the 2D band has an asymmetric shape and was found to be composed of two Lorentzian components. The peak positions of the TD and GF templates are located at 2,753 and 2,751 cm −1 , respectively. However, the spectra of the C 60 /TD and C 60 /GF FLG samples were dramatically changed compared with those before C 60 deposition, as shown in Fig. 3b,c . The first noticeable variation is a strong enhancement of the G band that was observed in both the C 60 /TD and C 60 /GF samples ( Fig. 3b–d ). The second is the enhancement of the 2D band intensity, which becomes comparable to that of G band intensity and is now a symmetric, single Lorentzian peak. The third difference is the 2D band peak shift to lower wavenumber from 2,753 to 2,727 cm −1 for C 60 /TD and from 2,751 to 2,703 cm −1 for 30 min C 60 deposition for C 60 /GF. The red shift of the 2D peak position from Bernal-stacked template graphene might be due to the decrease in interlayer interaction in TG. Similar behaviour of the 2D peak was observed between twisted graphene and Bernal-stacked bilayer graphene grown by CVD [16] . We also observed a blue shift of the 2D peak position between monolayer graphene and turbostratic graphene possessing monolayer graphene behaviour as shown in Supplementary Fig. 1 . The observed blue shift was ~19 and 6 cm −1 , respectively. Further detail is available in Supplementary Note 1 . It agrees well with previously reported results in artificially twisted CVD grown graphene layers [21] . Also the FWHM of 2D band became narrower compared with that of the Bernal-stacked template, from 117 to 54 cm −1 for C 60 /TD and from 111 to 43 cm −1 for C 60 /GF. This narrowing might be attributed to the reduction of interlayer coupling in our TG graphene. Interlayer interaction modifies the electronic band structure and the Raman properties. In strongly interacting AB-stacked Bernal graphene, the 2D/G ratio is lower than unity and the 2D peak is typically located at ~2,750 cm −1 . For the noninteracting graphene layers, one would expect that the Raman behaviour should be the same as for monolayer graphene where the 2D peak is typically located below 2,700 cm −1 and the 2D/G ratio is larger than unity. Weakly interacting graphene layers such as graphene on C-face SiC exhibit a 2D peak located between those of monolayer and AB-stacked graphene. A G peak enhancement (comparable to 2D peak) is also observed [22] . Previous Raman studies on TG have attributed a narrowing and intensity increase of the 2D peak to interlayer coupling and a modified electronic band structure [16] , [21] . Similar behaviour observed in our TG structures suggests that an interlayer interaction still exists as well. Raman mapping over a 0.8 mm × 0.8 mm area with 50 μm steps was performed on a C 60 /GF sample with GF growth for 20 min at 1,300 °C followed by C 60 deposition for 60 min at 1,400 °C. The 2D peak position and its FWHM were within the ranges ~2,710.5±0.38 cm −1 and ~48.3±2.7 cm −1 , respectively. The D/G ratio ranged within ~0.18±0.04 over the surface. The small D/G ratio value and its narrow variation indicate that twisted graphene with a low defect density was grown over the whole surface. Figure 3: Raman studies for graphene layer stacking order. Raman spectra of TD template (blue colour in a ) and C 60 /TD FLG sample (red colour in a ). inset) spectrum with SiC signal subtracted. 2D band of TD template has two Lorentzian components (black coloured curves), indicating Bernal stacking structure. ( b ) C 60 /TD FLG spectrum is composed of a single Lorentzian peak, indicating non-Bernal-stacked structure. Inset) spectrum with SiC signal subtracted. ( c , d ) Variation of Raman C 60 /GF FLG spectra as a function of C 60 deposition time. A single Lorentzian 2D band was observed for all samples studied. Black solid curves represent the fitted curve. ( e ) Comparison of GF template before and after thermal annealing for 30 min at 1,400 °C. Inset) curve fitting of 2D band of GF template sample. Full size image As the C 60 deposition is a high temperature (1,400 °C) process, the effect of temperature on rotational faults was examined. A GF template sample annealed for 60 min at 1,400 °C in the MBE growth chamber shows that there is no significant variation between the samples with and without annealing. Both have a high D/G peak ratio, a broad 2D band and multi-component of 2D bands. Therefore, we confirm that the observed twist is not induced by the temperature alone but rather by the C 60 deposition. Transport measurement and bandgap opening The transport characteristics of a C 60 /GF sample were evaluated by both I – V and temperature-dependent Hall effect measurements. It is worth noting that no gating voltage was applied in either experiment and that the bias voltage in the I – V measurements was applied through the CAFM (conductive atomic force microscopy) tip in a source-drain configuration. The I – V measurements were conducted at room temperature (RT). The red- and wine-coloured curves in Fig. 4a present the I – V curves of graphene directly grown by GF and C 60 on SiC, respectively, and show linear characteristics typical of zero bandgap graphene. However, twisted graphene (C 60 /GF) shows strong nonlinear I – V characteristics, which are commonly observed in graphene nanoribbons with a bandgap [23] , [24] . Han et al . [23] determined the transport gap from the width of the Δ V =0 region of their plot of d I /d V versus V . Similarly, we estimated the bandgap from where the differential conductance (d I /d V )≈0 as shown in Fig. 4b , which results in a gap of ~0.5 V. The I – V measurements at the different sample locations showed similar nonlinear I – V characteristics but with a gap in range from 0.2 to 0.5 V. It is well known that d I /d V versus V measurements can be affected by a variety of factors such as contact resistance, gating capacitance and so on, which can result in an overestimated bandgap size. However, the fact that nonlinear characteristics were only observed in C 60 /GF graphene suggests that Δ V ≈0 is correlated to the bandgap in TG. The existence of the bandgap has been further verified from the observation of thermal activation in the transport properties [24] , which is clearly seen in the high temperature carrier concentration and conductivity data shown in Fig. 4c . The temperature dependence of the conductivity in semiconducting graphene nanoribbons has been explained by invoking three different activation processes, thermally activated excitation across the gap, nearest neighbour hopping (NNH) and variable range hopping [23] . The best fits to our conductivity data gave only bandgap excitation and NNH without variable range hopping. This fitting well describes the measured conductivity (inset of Fig. 5c ) and results in a bandgap of ~80 meV. It should be noted that our low temperature carrier concentration data cannot be explained by hopping conduction. The difference in bandgaps from thermal activation and I – V measurements may be due to the fact that CAFM probes a small local region of the sample while our transport measurements are made over the whole 1 cm × 1 cm sample and thus average over the variations in the I – V measurements reported above. Nonetheless, the observed insulator state in the I – V measurements and the thermal activation experiments strongly support the existence of a bandgap in our C 60 /FG twisted graphene structure. 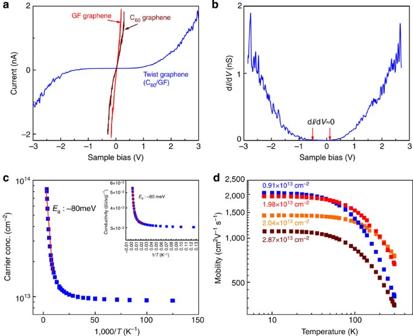Figure 4: Observation of intrinsic electronic bandgap in twisted graphene. Transport measurements on TG graphene grown by C60(flux: 1.6 × 10−7Torr) on GF (a)I–Vcurves from GF, C60and C60/GF TG graphene. (b) The dI/dVfor C60/GF TG graphene. (c) Temperature dependence carrier concentration obtained by Hall measurement. The solid curve is an aid to the eye to show activation behaviour. Inset: temperature-dependent conductivity. The solid colour line in inset plot is the curve fitted by band excitation and NNH conduction. (d) Temperature-dependent mobility for four different epitaxial TG samples. The carrier concentration value at each curve corresponds to the measured concentration at 10 K. Figure 4d presents the temperature dependence of the mobility for different carrier concentrations. The carrier type was p-type for the entire temperature region. The bare GF template (without C 60 deposition on it) had a high resistance (16 KΩ□ −1 ) and low mobility (62 cm 2 V −1 s −1 ). However, a strong enhancement of the electrical properties was observed on the C 60 /FG twisted graphene. The mobility at RT and 10 K are 400 and 2,050 cm 2 V −1 s −1 , respectively. As the temperature increases, the mobility monotonously decreases. This behaviour was not observed in FLG where the mobility is inversely proportional to temperature. Monolayer and quasi free-standing graphene exhibit a very weak temperature dependence to the mobility [16] , [25] . Similar behaviour was observed in the semiconductor MoS 2 (ref. 26 ). In the insulating state, Radisavljevic and Kis [26] observed strong temperature dependence at high temperatures and saturation of the mobility at low temperatures. In semiconductor materials, the mobility is limited by electron–phonon scattering and has the relation of μ ≈ T − α at high temperatures. Our C 60 /GF samples showed an α in the range from 1.76 to 2.0. A temperature independent mobility indicates that Coulomb scattering from charged impurities is not the dominant scattering mechanism at low temperature. The mobility showed an inverse proportionality to carrier concentration ( μ ≈1/ n ) at low temperature ( Fig. 4d ). Figure 4: Observation of intrinsic electronic bandgap in twisted graphene. Transport measurements on TG graphene grown by C 60 (flux: 1.6 × 10 −7 Torr) on GF ( a ) I – V curves from GF, C 60 and C 60 /GF TG graphene. ( b ) The d I /d V for C 60 /GF TG graphene. ( c ) Temperature dependence carrier concentration obtained by Hall measurement. The solid curve is an aid to the eye to show activation behaviour. Inset: temperature-dependent conductivity. The solid colour line in inset plot is the curve fitted by band excitation and NNH conduction. ( d ) Temperature-dependent mobility for four different epitaxial TG samples. 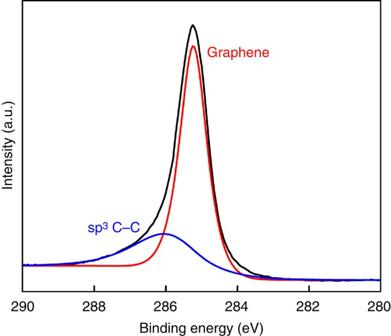Figure 5: Observation of sp3C–C bonding in twisted graphene. XPS C1s core level spectrum of epitaxial TG (C60: 2.5 × 10−7Torr). The fitting was done with a combination of Gaussian and Lorentzian peaks. The carrier concentration value at each curve corresponds to the measured concentration at 10 K. Full size image Figure 5: Observation of sp 3 C–C bonding in twisted graphene. XPS C1s core level spectrum of epitaxial TG (C 60 : 2.5 × 10 −7 Torr). The fitting was done with a combination of Gaussian and Lorentzian peaks. Full size image Observation of sp 3 interlayer C–C bonding Mele [8] proposed that the Dirac cones of TG are directly coupled across any commensurate rotation. The low energy band structure strongly depends on the sublattice parity. Even and odd sublattice exchange result in gapped materials and metallic graphene, respectively. Muniz and Maroudas [4] , [5] recently predicted that introducing interlayer C–C sp 3 bonding between pairs of graphene planes rotated with respect to each other generates defects in localized sp 3 C–C bonds and causes symmetry variations in graphene crystal structures. As a result, a bandgap as wide as 1.2 eV could open and that the band structure will be strongly dependent on the density and spatial distribution of the interlayer C–C sp 3 bonds. To check the existence of sp 3 C–C bonding, we performed XPS. As shown in Fig. 5 , our XPS measurements showed that the C1s peak consists of two component peaks located at 285.2 and 286 eV, respectively. The lower binding energy peak (285.2 eV) corresponds to graphene C–C sp 2 bonding. Díaz et al . [27] reported that the peak of sp 3 C atoms in carbon films shifts to higher energy and the energy difference ΔE between sp 2 and sp 3 C atoms is ~0.9 eV. This energy difference well agrees with our measurements (0.8 eV). Therefore, the peak at 286.3 eV can be attributed to sp 3 C–C bonding carbon. The sp 3 C–C interlayer bonding has been experimentally observed in graphite and carbon nanotubes modified by electron irradiation [28] , femtosecond laser excitation [29] and thermal treatment [30] without chemical functionalization. In addition, quantum molecular dynamics calculation have evidenced the existence of interlayer sp 3 C–C bonding between graphene layers contained defects such as vacancies and interstitials [31] . In our case, the formation of sp 3 hybridized carbons between layers of graphene becomes possible as carbon sources of thermally decomposed fullerene (C 60 ) gather near vacancy defects in existing template graphene layer. The presence of vacancies in template graphene can be confirmed by the detection of Raman D peak as shown in Fig. 3a because point defects such as vacancies is the only Raman active defect among various structural defects, while charged impurities, intercalants and strain are Raman inactive [32] . The appearance of Raman D suggests the existence of point defects such as vacancies in our template graphene. The necessary condition for this conjecture is that both decomposed fullerene source and point defects in the template graphene involve active carbons along the edge, which often allows a covalent bonding between active carbons aligned along the out-of-plane direction of the template graphene layer. The stability of such interlayer bonding should critically depend on the size of the vacant sites defect. An interlayer bonding over a single vacant site can exist temporarily as part of a transient configuration, which would disappear eventually as the new layer of carbon atoms surrounding the interlayer bonding relax into graphene structure. However, multiple interlayer bonding formed over sizeable vacancy sites has a high probability to remain as a localized amorphous domain of several carbon atoms kinetically jammed near the existing defects. To further support this conjecture, we performed growth simulations using self-consistent charge density functional tight binding molecular dynamics [33] , which allows quantum calculations of DFT accuracy in realistic simulations involving a large number of carbon atoms [34] . As fullerene molecules thermally decompose, various carbon structures of different molecular weight are available near the template graphene. We tested cleaved fullerenes and carbon trimers as two representative carbon sources after fullerene decomposition. Those carbon sources are added on the template graphene layer with both pristine graphene and vacancy defect where three or four carbon atoms are missing from otherwise pristine graphene. On pristine graphene, the supplied carbon molecules float over the graphene surface and merge into large carbon molecules. With this configuration, we do not observe any interlayer sp 3 C–C bonds ( Supplementary Fig. 2 ). On the graphene with vacancies, however, the growth kinetic becomes entirely changed. For both cleaved fullerenes and trimers cases, the interlayer bonding involving multiple sp 3 hybridized carbon is found near the vacancy defects of the template graphene as shown in Fig. 6 . Those interlayer C–C bonds involving sp 3 carbons were stable up to nanosecond at 1,000 K, and did not break during further energy minimization steps after MD simulations. When a further minimization is performed from the configuration of Supplementary Fig. 3b , the bonding configuration did not change at all. The free energy of this further minimized final state ( Supplementary Fig. 3b ) is 19.8 eV (0.14 eV per atom) lower than that of the initial state ( Supplementary Fig. 3a ). Further details of the simulations method and results are available in Supplementary Note 2 . From the modelling work, we could conclude that sp 3 interlayer C–C bonds connecting adjacent graphene layers become highly possible due to the nature of our growth method. That is, the graphene growth by external carbon molecules could be an alternative way to form interlayer carbon bonds into multilayer graphene without any ex situ chemical functionalization such as hydrogenation or fluorination [35] . 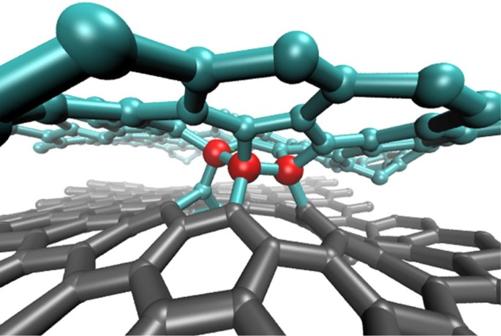Figure 6: Snapshot of an epitaxial growth molecular dynamics simulation using self-consistent charge density functional tight binding. Carbon trimer molecules are used as the growth source material on template graphene layer with vacancy defects. Grey-coloured atoms and bonds represent template graphene layer. Cyan-coloured atoms and bonds are newly grown graphene layer after growth simulation with trimer carbon source molecules. Red-coloured atoms show sp3hybridized interlayer carbons. Further information is available in theSupplementary Note 2. Figure 6: Snapshot of an epitaxial growth molecular dynamics simulation using self-consistent charge density functional tight binding. Carbon trimer molecules are used as the growth source material on template graphene layer with vacancy defects. Grey-coloured atoms and bonds represent template graphene layer. Cyan-coloured atoms and bonds are newly grown graphene layer after growth simulation with trimer carbon source molecules. Red-coloured atoms show sp 3 hybridized interlayer carbons. Further information is available in the Supplementary Note 2 . Full size image If the sp 3 C–C bonding observed in our TG sample ( Fig. 5 ) is related to interlayer linking, the concentration of sp 3 C–C bonding should increase with the thickness of the graphene layer. As C 60 deposition time increases from 1 to 30 min, the atomic concentration of sp 3 bonding increases from 7.25 at% to 27.54 at%. Therefore, we conclude that the sp 3 bonds result from interlayer C–C bonding. With this increase in the concentration of sp 3 C–C bonding, we observed the bandgap increased from 35 to 80 meV, which agrees with the monotonic increase of bandgap size with increasing sp 3 C–C bonds density in the predication of Muniz and Maroudas [4] , [5] . The bandgap size was estimated by the fitting of the temperature-dependent resistivity data with thermal activation and NNH conduction model. We have demonstrated that epitaxial TG with high mobility can be fabricated by C 60 CMBE deposition of graphene on pre-grown template graphene. Furthermore, this TG has a bandgap that we attribute to the rotational stacking faults and the formation of sp 3 interlayer C–C bonding. Our results are in agreement with the theory of Muniz and Maroudas. The size of the experimentally demonstrated intrinsic bandgap is determined by the modification of rotational stacking between graphene layers and the density of interlayer C–C bonding. Twisted graphene growth Epitaxial graphene was grown on chemical–mechanical polished on-axis SiC (0001) substrates by carbon molecular beam epitaxy in a high temperature molecular beam epitaxy system. The SiC substrate was ex situ cleaned with acetone and methanol, followed by a 10% HF dip to remove any native oxide. The carbon molecular beam was obtained from two different sources. C 60 was used with a conventional effusion cell to provide a uniform carbon flux. The carbon flux was measured with an ion-gauge. As a second carbon source, a pyrolytic graphite filament was used simultaneously as both the carbon source and the substrate heater by inverting the sample in the open-back substrate holder. The template graphene samples were grown by TD of SiC for 30 min. at 1,400 °C under a UHV environment and CMBE using a heated GF carbon source at 1,300 °C. C 60 was directly deposited to grow the additional graphene layers on the template by CMBE method. The substrate had to be removed from the chamber and remounted to switch from the GF to the C 60 sources. C 60 deposition was performed on TD graphene without remounting the substrate. Note that, separate template samples were used for each C 60 growth and for template alone characterization. ARPES measurement High-resolution ARPES data were taken at BL10.0.1 of the Advance Light Source at 15 K using photon energy of 50 eV. The vacuum was better than 3 × 10 −11 Torr and energy resolution was 23 meV. For ARPES measurement, the template was grown for 5 min at 1,300 °C with the GF carbon source, followed by C 60 deposition for 60 min at 1,400 °C. This template growth condition results in nominally monolayer thick graphene. Transport and Raman measurement I – V measurement was taken by Asylum Research Cypher scanning microscopy system at RT. Raman measurements were performed with a Renishaw InVia Reflex μRaman System with 514 nm wavelength excitation at RT. The laser beam was focused with × 100 objective lens to obtain 1 μm spot size. The temperature-dependent conductivity and Hall measurements were performed on 1 cm × 1 cm square samples with indium contacts at the four corners without any other processing using standard DC techniques. How to cite this article : Park, J. et al . Observation of the intrinsic bandgap behaviour in as-grown epitaxial twisted graphene. Nat. Commun. 6:5677 doi: 10.1038/ncomms6677 (2015).